Negative emissions physically needed to keep global warming below 2 °C To limit global warming to <2 °C we must reduce the net amount of CO 2 we release into the atmosphere, either by producing less CO 2 (conventional mitigation) or by capturing more CO 2 (negative emissions). Here, using state-of-the-art carbon–climate models, we quantify the trade-off between these two options in RCP2.6: an Intergovernmental Panel on Climate Change scenario likely to limit global warming below 2 °C. In our best-case illustrative assumption of conventional mitigation, negative emissions of 0.5–3 Gt C (gigatonnes of carbon) per year and storage capacity of 50–250 Gt C are required. In our worst case, those requirements are 7–11 Gt C per year and 1,000–1,600 Gt C, respectively. Because these figures have not been shown to be feasible, we conclude that development of negative emission technologies should be accelerated, but also that conventional mitigation must remain a substantial part of any climate policy aiming at the 2-°C target. Out of the four representative concentration pathways (RCPs) assessed by the Intergovernmental Panel on Climate Change (IPCC), RCP2.6 is the only one that likely limits global warming to <2 °C above preindustrial levels [1] . Following such a scenario needs a strong reduction in the net amount of fossil CO 2 released into the atmosphere by humankind [2] , [3] . This reduction can be achieved either by consuming less fossil fuels—and thus by producing less CO 2 molecules—or by capturing more of the human-produced CO 2 , through immediate capture at the site of production, direct removal of carbon dioxide from the atmosphere, or engineered enhancement of natural carbon sinks. Here we call the first option (less CO 2 production) ‘conventional mitigation’ and the second option (more CO 2 capture) ‘negative emissions’. This definition of negative emissions does not distinguish whether carbon dioxide is captured on site or removed from the free atmosphere. It is motivated by our goal of discussing future requirements for technologies; here we discuss requirements for technologies that do not currently exist at a large scale. However, a few of these technologies are at the stage of pilot projects. We note that the definition of ‘mitigation’ by IPCC WG3 encompasses both our conventional mitigation and negative emissions [4] . Our definition of negative emissions also differs from that of ‘carbon dioxide removal’ by IPCC WG1, which is restricted to the removal of CO 2 from the free atmosphere and therefore excludes on-site carbon capture from fossil-fuel power plants [5] . As part of the current debate on the role negative emissions might play in reaching the 2-°C target [6] , [7] , [8] , [9] , [10] , [11] , we hereby quantify the trade-off between conventional mitigation and negative emissions in the extended RCP2.6. We use a three-step approach to do so. First, we take fossil CO 2 emission trajectories estimated to be compatible with this scenario using Earth system models (ESMs). Second, we make assumptions about maximum feasible pathways of conventional mitigation, covering a wide range of possible futures. Third, calculating the mass balance for each of these pathways we deduce the gross negative emissions needed to be compatible with the RCP2.6 scenario. The ultimate product of our study is an abacus where one can make assumptions on future conventional mitigation and read the negative emission requirements—and associated uncertainty—compatible with maintaining global warming below 2 °C, as estimated by state-of-the-art ESMs. Our results suggest that negative emissions are needed even in the case of very high mitigation rates, but also that negative emissions alone cannot ensure meeting the 2-°C target. Emissions compatible with RCP2.6 RCPs are scenarios defined as trajectories of greenhouse gas concentrations [2] used to make climate change projections [1] . With global coupled carbon–climate models, they can also be used to estimate time series of fossil-fuel CO 2 emissions compatible with the trajectories. Indeed, given a prescribed trajectory of atmospheric CO 2 and the simulated changes in oceanic and terrestrial carbon reservoirs induced by changes in atmospheric CO 2 and climate, the so-called ‘compatible’ fossil-fuel emissions can be deduced by mass conservation of the element carbon [5] , [12] . In a given year, compatible emissions are positive if the total carbon stock of the atmosphere–ocean–land system increases, and negative if it decreases [12] (see also Methods). Here, we take estimates of fossil-fuel emissions compatible with RCP2.6 from the following: 11 three-dimensional ESMs used in the Fifth IPCC report [5] , [12] ; an ensemble of simulations made with an Earth system model of intermediate complexity named JUMP-LCM (ref. 13 ); another ensemble produced with a simple carbon–climate model named OSCAR (ref. 14 ). Emissions from industrial processes are included but not those from land-use and land-cover change (see Methods). Estimates by ESMs are only available over the 21st century while the others follow the scenario’s extension up to 2300 (ref. 2 ). 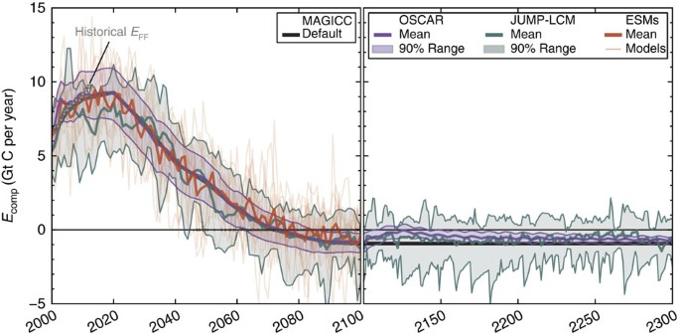Figure 1: Fossil-fuel emissions estimated to be compatible with RCP2.6. Estimates by ESMs, ensembles by JUMP-LCM and OSCAR, as well as the default fossil-fuel emissions for RCP2.6 are shown. The latter are compatible with the simple carbon–climate model MAGICC6 over 2000–2100 (ref.2). Historical emissions from fossil-fuel burning (EFF) are also provided18. Figure 1 shows these compatible emissions. During the 21st century, all the average trajectories are very close to each other, with <10% difference in terms of cumulative emissions. After 2100, however, these differences increase (see the discussion in the Methods section). The uncertainty in the compatible emissions shown in Fig. 1 stems from the different representations of carbon-cycle processes and climate–carbon feedbacks in the models. Figure 1: Fossil-fuel emissions estimated to be compatible with RCP2.6. Estimates by ESMs, ensembles by JUMP-LCM and OSCAR, as well as the default fossil-fuel emissions for RCP2.6 are shown. The latter are compatible with the simple carbon–climate model MAGICC6 over 2000–2100 (ref. 2 ). Historical emissions from fossil-fuel burning ( E FF ) are also provided [18] . Full size image Disentangling net and gross emissions The key point about these compatible emissions is that they are deduced from carbon–climate model simulations: they only reflect responses of the natural systems and do not contain information on how they are achieved by human societies. Therefore, these emissions are global net emissions and they can be broken down into gross positive and gross negative emissions. If there was no constraint of any sort, one could imagine ever-growing positive emissions from fossil-fuel burning, compensated by even stronger negative emissions needed to meet the trajectories shown in Fig. 1 . In this study, we define a series of ‘mitigation floors’, which are assumed trajectories of maximum conventional mitigation of fossil-fuel emissions that could be achieved. This concept of mitigation floor is used to encompass technical, economic, sociopolitical inertia [15] , [16] and limits [17] in reducing the gross positive fossil CO 2 flux (that is, in reducing the consumption of fossil fuel). It is the maximum potential mitigation at a given time. Thence, as long as the mitigation floor is lower than compatible emissions, there is no physical need for negative emissions, since reaching compatible emissions can be achieved through conventional mitigation only. However, if the floor is greater than compatible emissions, negative emissions are a physical requirement (see Methods). 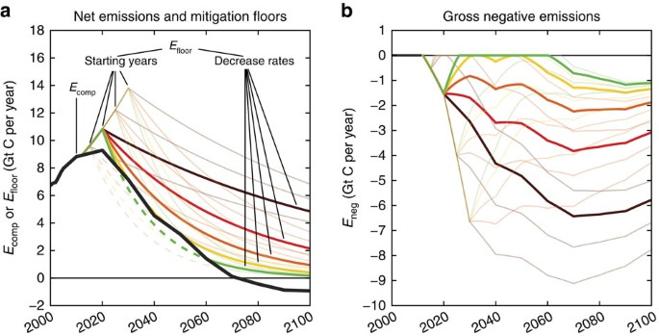Figure 2: Illustration of the default mitigation floors and corresponding gross negative emissions. (a) Only one compatible emissions trajectory (Ecomp) and all the possible mitigation floors (Efloor) for this trajectory. (b) In a given year, the requirement for negative emissions (Eneg) corresponds to the gap between the mitigation floor and compatible emissions, should there be any. Figure 2 presents the several mitigation floor assumptions of our study. In 2012, compatible emissions are taken as the reference. After that, the floor follows a business-as-usual increase of +2.46% per year, as per fossil-fuel emissions over the 2007–2012-period [18] . Then it starts decreasing at various points in time: 2015, 2020, 2025 or 2030. These decreases are assumed to occur exponentially at various rates: −5%, −4%, −3%, −2% or − 1% per year. The choice of an exponential shape for mitigation floors is motivated by them being defined as ‘trajectories of maximum conventional mitigation’. Consistently, we assume the most effective mitigation options will be implemented first, leaving less effective ones to be implemented afterwards. This leads to exponential shapes of mitigation floors: the marginal effectiveness of mitigation is decreasing with time. We acknowledge, however, that arguments can be made for other shapes, and those alternative shapes are discussed hereafter. Figure 2: Illustration of the default mitigation floors and corresponding gross negative emissions. ( a ) Only one compatible emissions trajectory ( E comp ) and all the possible mitigation floors ( E floor ) for this trajectory. ( b ) In a given year, the requirement for negative emissions ( E neg ) corresponds to the gap between the mitigation floor and compatible emissions, should there be any. Full size image The rates of conventional mitigation are taken to cover a wide range of possible futures (and numerous positive emission trajectories from integrated assessments fall in their range; see Supplementary Fig. 1 ). For instance, our rates are comparable to the following: the decreased rate of emissions committed by the lifetime of emitting infrastructures that may range, depending on the assumptions, from −5.7% per year to −3.2% per year over 2010–2050 (refs 15 , 19 ); the observed historical decarbonation rate of −4.6% per year during the French nuclear program of 1980–1985 (ref. 20 ); the average 2008–2020 mitigation rate of −1.3% per year pledged by the United States needed to reach in 2020 −17% of emission compared with 2005, or of −1.0% per year pledged by the European Union to reach in 2020 −20% compared with 1990 (ref. 20 ). Note that all these rates are mean annual rates of change: they are thus strictly comparable to our exponential rates, and fairly comparable to linear rates (later used for alternative mitigation floors). This justifies the `fairly comparable' rates. We use that kind of stylized economic pathways to explore ‘what-if’ scenarios without making complex and debated [21] , [22] , [23] assumptions as it is done for integrated assessments. We hereby provide physically based estimates of negative emission requirements in the form of a table whose inputs are our two simple parameters: the starting year and the rate of decrease of the mitigation floor. That table’s outputs are condensed in Fig. 3 . 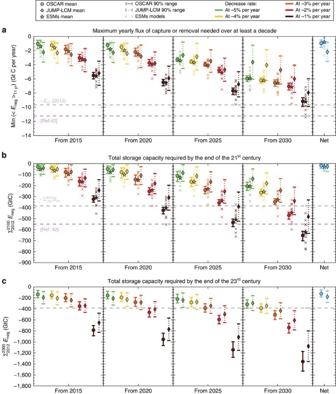Figure 3: Negative emission requirements for our default mitigation floor assumptions. (a) The maximum yearly flux of carbon capture or removal required over at least a decade. (b) The cumulative carbon captured or removed by the end of the 21st century and (c) the cumulative capture or removal by the end of the 23rd century. Each panel is broken down into one sub-panel per starting year of decrease of the mitigation floor. Inside each sub-panel, colours refer to rates of decrease (from −5 to −1% per year, from left to right, respectively) and symbols to models. ‘90% ranges’ correspond to the range between the 5th and the 95th percentiles. Estimates when no mitigation floor is considered (that is, of net negative emissions) are shown in the right-most sub-panels. The opposite of historical emissions from fossil-fuel burning18(EFF) and the gross negative emissions in the ‘original’ RCP2.6 (ref.42) are also provided for comparison (dashed horizontal grey and magenta lines, respectively). Figure 3: Negative emission requirements for our default mitigation floor assumptions. ( a ) The maximum yearly flux of carbon capture or removal required over at least a decade. ( b ) The cumulative carbon captured or removed by the end of the 21st century and ( c ) the cumulative capture or removal by the end of the 23rd century. Each panel is broken down into one sub-panel per starting year of decrease of the mitigation floor. Inside each sub-panel, colours refer to rates of decrease (from −5 to −1% per year, from left to right, respectively) and symbols to models. ‘90% ranges’ correspond to the range between the 5th and the 95th percentiles. Estimates when no mitigation floor is considered (that is, of net negative emissions) are shown in the right-most sub-panels. The opposite of historical emissions from fossil-fuel burning [18] ( E FF ) and the gross negative emissions in the ‘original’ RCP2.6 (ref. 42 ) are also provided for comparison (dashed horizontal grey and magenta lines, respectively). Full size image Negative emissions required in RCP2.6 The maximum yearly flux of negative emissions that needs to be sustained over at least a decade is shown in Fig. 3a . Across all our mitigation floor assumptions, this maximum flux varies tenfold. In our best-case assumption (decrease starting in 2015 at a rate of −5% per year), this value ranges from 0.5 to 3 Gt C per year (see Methods for how ranges are obtained). In our worst-case assumption (-1% per year starting in 2030), it goes from 7 to 11 Gt C per year. The latter value is the same order of magnitude as global CO 2 emission from fossil-fuel burning in 2012 (ref. 18 ). When taken as a function of the mitigation floor decrease rate, this maximum flux of removal is nonlinear: if the decrease rate (that is, the rate of society’s transformation) is for instance halved, then the maximum flux of CO 2 removal required is more than doubled. Thus, any efforts put into mitigation would be more than compensated by an alleviation of the requirement for negative emissions (in terms of carbon dioxide, not of economic or risk trade-off analysis). The time at which this maximum flux has to be achieved can vary greatly but, generally speaking, the longer we wait to start mitigation, the sooner the maximum flux is needed ( Supplementary Fig. 2 ). Also, given the limited potential of each negative emission technology [5] , a combination of several technologies will probably be needed to deliver this maximum yearly flux. The cumulative amount of carbon that needs to be captured on site or from the atmosphere is also a key value, because this carbon somehow has to be stored. Figure 3 shows how much carbon storage is needed by 2100 ( Fig. 3b ) and by 2300 ( Fig. 3c ). In our best-case assumption, 25–100 and 50–250 Gt C of storage capacity are needed by the end of the 21st and 23rd century, respectively. In our worst-case assumption, there is a need for a capacity of 450–800 by 2100, and 1,000–1,600 Gt C by 2300. Ending the study in 2300 rather than 2100 roughly doubles the amount of carbon storage required. This total amount of captured carbon dioxide, be it up to 2100 or 2300, is a nonlinear function of the decrease rate of the mitigation floor and of the starting year of decrease. Thus, any reduction or postponing of the effort in mitigation increases even more the total amount of CO 2 that has to be captured and stored. Globally, depleted oil and gas reservoirs and coal seams are estimated to have a storage capacity of 300–350 Gt C, and saline aquifers a capacity of 1,100–6,300 Gt C (ref. 24 ), which is more than all of our requirement estimates. However, these capacity values do not account for technical feasibility, economic costs and social acceptability, which indicates the actual storage capacity is likely to be lower. Alternative mitigation floors Given that the mitigation floor is so crucial to the study, we investigated three alternative shapes for it (illustrated in Supplementary Figs 3 and 4 ). The corresponding negative emission requirements are detailed in Supplementary Figs 5–8 , where one can see that changing the mitigation floor’s shape does not drastically change the qualitative conclusions of this study. It does change, however, the quantitative estimates of negative emission requirements, and those quantitative changes are summarized hereafter. We also note that all these assumed shapes of mitigation floors are idealized. There is no reason that actual future trajectories of mitigation follow exactly those shapes: they will vary accordingly to the economic, technological and sociopolitical context of the moment. First, we looked at a flat transition (instead of a business-as-usual increase) between 2012 and the starting year of decrease of the floor. This shape of the mitigation floor could represent, for instance, a transition period during which global CO 2 production would be stabilized before being actually reduced. Comparatively to the default shape, this one ignores the difficulties in the short-term transition to an effectively decreasing mitigation pathway. This short-term transition could be studied with integrated assessment models (IAMs) [25] , [26] . Whatever the assumed floor characteristics (starting year and rate of decrease), such a change in its shape reduces both maximum yearly and cumulative negative emission requirements by up to 60% in the case of slow mitigation starting late. Second, we considered a linear decrease of the mitigation floor (instead of exponential), which means that a constant amount of positive emission is mitigated each year, independently of the current level of emission. One could argue that this shape is a better choice to represent the first years of a mitigation trajectory than our default shape (it was used, for example, by Kriegler et al . [9] ). For all our mitigation floor characteristics, this change in shape reduces both the maximum flux and the storage needed by up to 50% in the case of rapidly decreasing floors. Since this shape of the mitigation floor does reach the asymptote of 0, the reduction is very pronounced when looking at the storage capacity in 2300. Third, we defined a ‘hard floor’ of 1 Gt C per year as being the lower limit of the mitigation floor (that is, the floor tends asymptotically towards this value, instead of towards zero in the default case). Adding such a hard floor increases the maximum flux requirement by ∼ 1 Gt C per year and the storage requirement by 1 Gt C for each year in the considered period. Hence, if it really were impossible to reduce anthropogenic CO 2 emission from fossil-fuel burning below that hard floor of 1 Gt C per year, an additional storage capacity of about 300 Gt C would be required by the end of the 23rd century. This value is comparable to the increase in storage capacity requirement if mitigation of fossil CO 2 emission were to be delayed by 15 years. When comparing our mass-balance estimates of gross negative emissions with those by IAMs, ours fall in the lower end of the range [7] , [8] , [9] , [27] , [28] (see also Supplementary Fig. 9 ). This logically follows our approach of always choosing conventional mitigation over negative emissions when the mitigation potential allows it (that is, when the mitigation floor is higher than the compatible emissions). Our approach thus provides a physical lower bound of negative emission requirements for a given mitigation potential. Conversely, in integrated assessments, negative emissions may be chosen over conventional mitigation at any time, depending on which is found more economical to develop under assumed costs and technological potentials. In our study, all the assumptions about technologies, costs and even sociopolitical systems are lumped together in the concept of the mitigation floor, rendering detailed socioeconomic analysis impossible. Another major difference with studies using IAMs is that ours rely on state-of-the-art Earth system models. Despite the drawback of having to set some drivers exogenously (see Methods), it allows a comprehensive assessment of the uncertainty related to the future response of the carbon–climate system. Figure 3 shows this uncertainty can be greater than the results between two different mitigation floor assumptions. It emphasizes that the uncertainty surrounding any policy decision related to negative emissions primarily comes from our lack of understanding of the future behaviour of the Earth system. Paradoxically, this high uncertainty is also one of the reasons why negative emissions may be needed in the future. The risk management function of negative emission technologies [29] would lessen the impacts of climate change if it were to run amok, because of unanticipated natural positive feedbacks. Furthermore, our study has ignored some physical processes, and negative emission requirements could actually be higher than we estimate. For instance, of all our models only two [12] ESMs include the restrictive effect of nitrogen limitation upon future land carbon sinks [30] . A reduction in future carbon sinks would reduce compatible emissions, and thus increase the need for negative emissions. Permafrost thawing, as a potential future source of carbon, is also not accounted for in our study, and it may similarly reduce compatible emissions [31] . Compatible emissions used here are restricted to the RCP2.6 land-use change scenario (see Methods). A future with more deforestation than in this scenario would see reduced compatible emissions through two mechanisms: increased CO 2 emissions from land-use change and loss of potential land carbon sink [32] . We also assumed no leakage of the storage reservoirs—such leakage could reduce compatible emissions as well. Finally, choosing additional climate targets other than the increase in global mean temperature (for example, limiting ocean acidification) may also reduce compatible emissions [33] and again increase gross negative emission requirements. The goal of this study was to discuss negative emission requirements, in the context of the 2-°C target, with an atypical but complementary approach: with Earth system models instead of IAMs. Although our physically oriented approach brought new results, especially regarding the quantification of physical uncertainties, we acknowledge that using the mitigation floor concept does not provide as much detail about the socioeconomic system as integrated assessments usually do (for example, about the evolution in energy services demands, about the share of specific technologies in the energy mix or about the energy efficiency improvements, in various sectors and regions). In other words, the strengths and weaknesses of the two approaches are in opposition with regard to the natural and anthropogenic systems. The next logical step is to couple both approaches to preserve their respective strengths. This would be achieved by fully integrating an ESM to an IAM and more specifically, an ESM complex enough to account for key nonlinear processes of the carbon-cycle and climate systems. Among those processes, we believe focus should be on the following: the biophysical effect of land-use change and land management [34] , especially since most low-carbon scenarios in IAMs rely on Bio-Energy and Carbon Capture and Storage (BECCS) (ref. 35 ); the climate-induced changes in natural emissions such as those from natural wetlands or permafrost [5] . This coupling between an IAM and a complex ESM would help discuss the feasibility of trajectories surrounding 2 °C and more importantly, it would help assess the risk associated with overshooting this target. To conclude, we find that negative emissions are required at significant levels (that is, >1 Gt C per year) to meet the 2-°C target, even for very aggressive mitigation floors. Given that negative emission technologies—both on-site capture and atmospheric removal—are still at an early stage of development [36] , [37] , this pleads in favour of developing (financial) mechanisms to put them on a technological learning trajectory [37] . But then, in all but the most optimistic cases, we also find negative emission requirements that have not yet been shown to be achievable: be it the yearly flux of combined capture and removal or the storage capacity. Following others [35] , [38] , [39] , this study suggests that negative emissions alone are unlikely to be the panacea that will limit global warming below 2 °C, and that conventional mitigation—that is, reduced consumption of fossil fuels—should remain a significant part of any climate policy aiming at this target. Models’ description The 11 ESMs whose results are taken for this study were all used in the IPCC Fifth Assessment Report [5] . JUMP-LCM is an Earth system model of intermediate complexity built to mimic the full ESM MIROC3, of which key parameters (such as climate sensitivity, diffusivity in the ocean, maximum photosynthetic rate and so on) were varied to represent the behaviour of C 4 MIP models as much as possible [13] . OSCAR v2.1 is a simple carbon–climate model whose modules are designed to emulate a range of sensitivities derived from model intercomparisons such as C 4 MIP or CMIP5 (refs 14 , 40 ). For the last two models, we take ‘constrained’ ensembles of compatible emissions that were compared and rated against observations of various climate variables [13] , [14] . The global mean temperature projections by the models are shown in Supplementary Fig. 10 , and their transient climate response to (cumulative) emissions are shown in Supplementary Fig. 11 . Compatible emissions Applying the constraint of global mass conservation, annual compatible fossil-fuel emissions ( E comp ) are calculated for all global carbon–climate models, as being equal to the annual variation of the natural carbon reservoirs: atmosphere ( C A ), ocean ( C O ) and land ( C L ): To estimate the change in carbon stocks of ocean and land, models were prescribed atmospheric CO 2 concentration following historical estimates up to 2005 and the RCP2.6 scenario and its extension afterwards [2] . Depending on the study [12] , [13] , [14] , however, other climate forcings (other greenhouse gases, short-lived species and natural forcings) were prescribed as concentrations or directly as radiative forcing, which is thus a source of discrepancy among the estimates of compatible emissions. Note that these non-CO 2 forcings do impact the estimates of compatible emissions through their effect on climate change, which then feeds back on the carbon cycle. The RCP2.6 land-use and land-cover change scenario [41] is also prescribed in all models, albeit only up to 2100. Thus, CO 2 emissions from land-use and land-cover change are accounted for in the compatible emission estimates, as they are part of the net change in land carbon storage C L (refs 5 , 12 ). Note also that the stop in the land-use change scenario in 2100 explains the small rebound of compatible emissions estimated by OSCAR. This rebound is stronger in OSCAR than in JUMP-LCM, because the former model includes an explicit book-keeping module to calculate CO 2 emissions from land-use and land-cover change [14] , [30] . Mitigation floors For each trajectory of compatible emissions, the reference ( E ref ) used for the mitigation floor ( E floor ) is taken as being equal to the average of annual compatible emissions over the 2010–2014-period for JUMP-LCM and ESMs (to account for interannual variability), and strictly equal to the 2012 value for OSCAR (no variability in this model). In a given year t , the mitigation floor that is assumed to start decreasing in the year t d at a negative rate r is formulated as: Negative emissions Finally, the required yearly negative emissions ( E neg ) are estimated as the difference between the mitigation floor and compatible emissions, only when the floor is above compatible emissions: For Fig. 3 , the maximum yearly flux of carbon removal is calculated with a moving average over 11 years, which broadly erases interannual variability and assumes that this flux would have to be sustained over at least a decade. The cumulative amount of carbon removed from the atmosphere is simply taken as the sum of negative emissions over the 2012–2100- or 2012–2300-periods. Ranges given in the text are from the ESMs when available. When results from the ESMs are not available (that is, for a storage capacity up to 2300), we calculate them using the mean value from OSCAR as best guess and the 90% range from JUMP-LCM as spread around the best guess. This is supported by the fact that (when comparison can be made) the mean from OSCAR is broadly in line with the mean from ESMs, and the 90% range from JUMP-LCM is also broadly in line with the spread among ESMs. How to cite this article : Gasser, T. et al . Negative emissions physically needed to keep global warming below 2 °C. Nat. Commun. 6:7958 doi: 10.1038/ncomms8958 (2015).